Stratonovich-to-Itô transition in noisy systems with multiplicative feedback Intrinsically noisy mechanisms drive most physical, biological and economic phenomena. Frequently, the system’s state influences the driving noise intensity (multiplicative feedback). These phenomena are often modelled using stochastic differential equations, which can be interpreted according to various conventions (for example, Itô calculus and Stratonovich calculus), leading to qualitatively different solutions. Thus, a stochastic differential equation–convention pair must be determined from the available experimental data before being able to predict the system’s behaviour under new conditions. Here we experimentally demonstrate that the convention for a given system may vary with the operational conditions: we show that a noisy electric circuit shifts from obeying Stratonovich calculus to obeying Itô calculus. We track such a transition to the underlying dynamics of the system and, in particular, to the ratio between the driving noise correlation time and the feedback delay time. We discuss possible implications of our conclusions, supported by numerics, for biology and economics. Mathematical models are often employed to predict the behaviour and evolution of complex physical, chemical, biological and economic phenomena. Often, more realistic mathematical models can be obtained by allowing for some randomness. In a dynamical system, for example, this randomness can be introduced by adding a noisy driving term, where a noise x t drives the evolution of the state y t of the dynamical system ( Fig. 1a ). Similar models have been employed to describe a wide range of phenomena, from thermal fluctuations of microscopic objects [1] and the evolution of stock prices [2] to the heterogeneous response of biological systems to stimuli [3] and stochasticity in gene expression [4] . 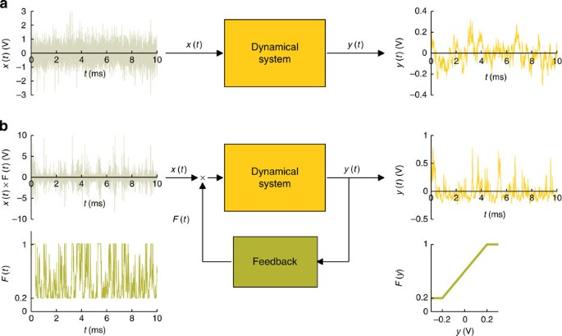Figure 1: Stochastic dynamical system without and with feedback. (a) Schematic representation of a stochastic dynamical system: the system’s statusy(t) evolves as the system is driven by a noisy inputx(t). (b) Same system with feedbackF(y(t)):x(t) is now modulated byF(y(t)) andy(t) is clearly affected. Figure 1: Stochastic dynamical system without and with feedback. ( a ) Schematic representation of a stochastic dynamical system: the system’s status y ( t ) evolves as the system is driven by a noisy input x ( t ). ( b ) Same system with feedback F ( y ( t )): x ( t ) is now modulated by F ( y ( t )) and y ( t ) is clearly affected. Full size image Intrinsically noisy phenomena are often modelled by stochastic processes, in particular, solutions of stochastic differential equations (SDEs) (see reference texts for a readable application-oriented introduction [5] and for a thorough mathematical treatment [6] , [7] ). An SDE is obtained by adding some randomness to a deterministic dynamical system described by an ordinary differential equation (ODE) [8] . The simplest form of an SDE is: where G ( y ) is a function representing the deterministic response of the system, W t is a Wiener process representing the stochastic driving and σ is a scaling constant representing the intensity of the noise. The term σ dW t is thus a mathematical model of the physical noise. In particular, any real process always has a correlation time τ >0, while dW t is strictly uncorrelated, that is τ =0; therefore, the smaller the τ of a real process, the better it is approximated by dW t (ref. 9 ). We remark that, under fairly general assumptions, Equation 1 with a given initial condition y 0 has a unique solution; this solution satisfies the integral equation y t = y 0 +∫ 0 t G ( y s )d s +σ W t (ref. 5 ). In many real phenomena, the system’s state further influences the driving noise intensity ( Fig. 1b ); for example, the volatility of a stock price may be altered by its actual value [10] or the expression of a gene may be regulated by the concentration of its products [4] . This multiplicative feedback F ( y ) leads us to consider an SDE with multiplicative noise: Unlike Equation 1, the integration of Equation 2 presents some difficulties because W t is a function of unbounded variation [5] . The stochastic integral , where and α ∈ (0,1), may lead to different values for different choices of α (refs 6 , 11 ). Common choices are: the Itô integral with α =0 (ref. 12 ); the Stratonovich integral with α =0.5 (ref. 13 ), and the anti-Itô or isothermal integral with α =1 (ref. 14 ). Alternative values of α may entail dramatic consequences ( Supplementary Note 1 ): for example, a Malthusian population growth model with a noisy growth rate can lead either to exponential growth ( α =0.5) or to extinction ( α =0) ( Supplementary Fig. S1 ); a logistic population growth model predicts very different long-term population size depending on α ( Supplementary Fig. S2 ); the expected return on a risky investment can be either larger ( α =0.5) or smaller ( α =0) than the one on a safe investment ( Supplementary Fig. S3 ); and a metastable physical system ( α =0.5) can turn into a bistable system ( α =0) ( Supplementary Fig. S4 ). Therefore, a complete model is defined by an SDE and the relative convention, which must be determined on the basis of the available experimental data [15] . If desired, one can change the convention, but only by adding an appropriate drift term at the same time. We emphasize that in the present article the coefficients of the equation do not change; it would also be possible to keep the Itô convention throughout and change the drift term accordingly as α varies [16] . Various preferences regarding the appropriate choice of α have emerged in various fields in which SDEs have been fruitfully applied. For example, α =0 models are typically employed in economics [5] and biology [17] , because of their property of ‘not looking into the future’, referring to the fact that, when the integral is approximated by a sum, the first point of each interval is used. α =0.5 naturally emerges in real systems with non-white noise, that is τ >0, for example, the SDEs describing electrical circuits driven by a multiplicative noise [18] , as explained mathematically by the Wong–Zakai theorem, which states that, if in Equation 2 the Wiener process is replaced by a sequence of smooth processes with τ →0, the resulting limiting SDE obeys the Stratonovich calculus [19] . Finally, α =1 naturally emerges in physical systems in equilibrium with a heat bath [20] , [21] , [22] . Other values of α have also been theoretically proposed [16] , [23] , [24] . From the modelling perspective the choice of the appropriate SDE-convention pair is of critical importance, especially when the model is subsequently employed to predict the system’s behaviour under new conditions. In this article, we experimentally demonstrate that the convention for a given physical system can actually vary under changing operational conditions. We show that the equation describing the behaviour of an electric circuit with multiplicative noise, which usually obeys the Stratonovich convention ( α =0.5) [18] , crosses over to obey the Itô convention ( α =0), as certain parameters of the dynamical systems are changed. This transition is continuous, going through all intermediate values of α . We relate this transition by an explicit formula to the ratio between τ and the feedback delay time δ , which are both non-zero in any real system. We mathematically demonstrate that this transition occurs for all delayed SDEs with multiplicative noise. Such transitions have the potential of dramatically altering a system’s long-term behaviour and, therefore, we argue their possibility should be taken into account in the modelling of systems with SDEs. System without feedback As a paradigmatic experimental realization of a noisy system, we consider an RC-electric circuit with resistance R =1 kΩ and capacitance C =100 nF; x t is the driving voltage (applied on the series RC) and y t the output voltage (measured on C) ( Fig. 2a ). In order to approximate a Wiener process, we will always use a driving noise with a correlation time much shorter than the typical relaxation time of the circuit, that is, . A detailed description of the circuit is given in the Methods. The output voltage y experiences an elastic restoring force with elastic constant k =1/ RC towards the y =0 equilibrium state, that is, the system behaves as a harmonic oscillator. 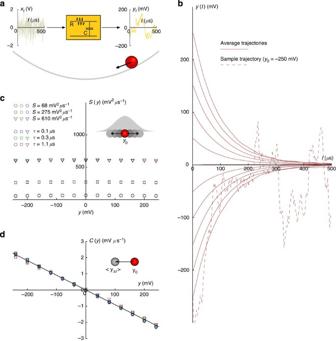Figure 2: Stochastic dynamical system without feedback. (a) In our experiments, we employ an RC electric circuit driven by a noisext; the system’s stateyteffectively experiences a harmonic restoring forceG(y)=−kywithk=1/RC. (b) Sample trajectory ofyt(τ=1.1 μs) with initial conditiony0=−250 mV (dashed line) and average of 1,000 trajectories for various initial conditions (solid lines). (c) DiffusionS(y) and (d) driftD(y) of the system’s state for various intensities and correlation times (τ) of the input noise.S(y) is proportional to the variance of the system state change (inset in (c)) andD(y) to its average (inset in (d)). The solid line in (d) represents the harmonic restoring forceG(y). Figure 2: Stochastic dynamical system without feedback. ( a ) In our experiments, we employ an RC electric circuit driven by a noise x t ; the system’s state y t effectively experiences a harmonic restoring force G ( y )=− ky with k =1/ RC . ( b ) Sample trajectory of y t (τ=1.1 μs) with initial condition y 0 =−250 mV (dashed line) and average of 1,000 trajectories for various initial conditions (solid lines). ( c ) Diffusion S ( y ) and ( d ) drift D ( y ) of the system’s state for various intensities and correlation times ( τ ) of the input noise. S ( y ) is proportional to the variance of the system state change (inset in ( c )) and D ( y ) to its average (inset in ( d )). The solid line in ( d ) represents the harmonic restoring force G ( y ). Full size image In order to understand qualitatively the behaviour of our system, in Fig. 2b we consider the evolution of y t for a given initial condition y 0 and τ=1.1 μs. The dashed line illustrates a sample trajectory for y 0 =−250 mV: at the beginning y t decays towards the equilibrium y =0 mV and, afterwards, oscillates around the equilibrium, clearly demonstrating its stochastic nature. Averaging several such trajectories, we obtain solid lines corresponding to different y 0 , which clearly shows that the average trajectory moves towards the equilibrium regardless of y 0 . The relevant SDE is Equation 1 with G ( y )=− ky and σ is the intensity of the noise, that is: where k >0. This equation has an explicit solution (the Ornstein–Uhlenbeck process) that, as in all cases with a constant σ (ref. 6 ), is independent of the choice of α and, therefore, the convention can be left undetermined. We determined the stochastic diffusion S ( y ) and the drift D ( y ) of this system as described in the Methods. The symbols in Fig. 2c represent the experimental values of S ( y ) for various σ and τ ; they clearly show that, for the system described by Equation 3, S ( y ) is a constant that depends only on the intensity of the input noise σ , that is, and not on τ . Figure 2d shows the deterministic response G ( y ) (solid line) and the experimental values of D ( y ) (symbols); the values of D ( y ) lay on the graph of G ( y ) independently of σ and τ . We note that the absence of dependence on τ for both S ( y ) and D ( y ) demonstrates that a white noise is a good model for the coloured driving noise used in our experiments, that is, with τ ≤1.1 μs. System with feedback Now we introduce a multiplicative feedback in the circuit as shown in Fig. 3a . This is achieved by multiplying the input noise by F ( y ). As shown in Fig. 3b , F ( y ) increases linearly between −80 mV and 160 mV and saturates to 0.2 V (1 V) for y <−80 mV ( y >160 mV). The details of the circuit with multiplicative feedback are given in the Methods. 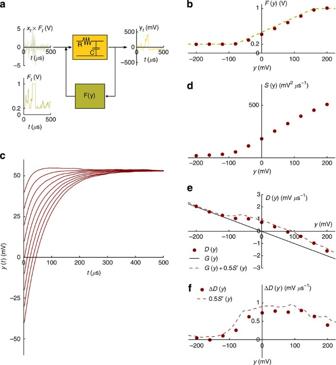Figure 3: Stochastic dynamical system with feedback. (a) Schematic representation of a stochastic dynamical system with multiplicative feedbackF(y): the driving noisext(τ=1.1 μs) is multiplied by a function of the system’s stateyt. (b) Nominal (dashed line) and experimentally measured (dots) feedback function used in our experiments. (c) Average of 1,000 trajectories for various initial conditions; there is a clear shift of the equilibrium in comparison with the case without feedback (Fig. 2d). (d) DiffusionS(y) (dots) and (e) driftD(y) (dots) of the system status. In (e), the solid line represents the harmonic restoring forceG(y) and the dashed lineG(y)+0.5S′(y). (f) Agreement between the noise-induced extra-drift ΔD(y) and 0.5S′(y). The relevant SDE is: Figure 3: Stochastic dynamical system with feedback. ( a ) Schematic representation of a stochastic dynamical system with multiplicative feedback F ( y ): the driving noise x t ( τ =1.1 μs) is multiplied by a function of the system’s state y t . ( b ) Nominal (dashed line) and experimentally measured (dots) feedback function used in our experiments. ( c ) Average of 1,000 trajectories for various initial conditions; there is a clear shift of the equilibrium in comparison with the case without feedback ( Fig. 2d ). ( d ) Diffusion S ( y ) (dots) and ( e ) drift D ( y ) (dots) of the system status. In ( e ), the solid line represents the harmonic restoring force G ( y ) and the dashed line G ( y )+0.5 S ′( y ). ( f ) Agreement between the noise-induced extra-drift Δ D ( y ) and 0.5 S ′( y ). Full size image whose properties cannot be inferred without additional assumptions, that is, an explicit specification of α is required in order for this SDE to be well-defined. For the case of an electric circuit driven by a coloured noise, that is, a stochastic process with a characteristic correlation time τ >0, the Stratonovich convention holds, as is expected theoretically from the Wong–Zakai theorem [19] and has been shown experimentally [18] . In fact, we see that the Stratonovich integral also describes the system in our case. When τ =1.1 μs, differently from the case without feedback ( Fig. 2b ), the average trajectories in Fig. 3c do not converge to y =0, but to y =50 mV. This shift of the equilibrium is a consequence of the non-uniformity of S ( y ) ( Fig. 3d ) due to the presence of a multiplicative feedback. We remark that S ( y ) is independent from the interpretation of the underlying SDE [25] . D ( y ) (symbols in Fig. 3e ) is also altered as a consequence of the multiplicative noise. In particular, D ( y ) is now different from G ( y ) (solid line in Fig. 3e ). The difference between the two is a noise-induced additional drift which is represented by the symbols in Fig. 3f . The relation between Δ D ( y ) and the variation of S ( y ), that is, , becomes evident considering the good agreement between Δ D ( y ) and 0.5 S ′( y ) (dashed line in Fig. 3f ). The prefactor 0.5 corresponds to the α of the Stratonovich interpretation of the SDE (4), which permits us to make sense of the experimentally observed data. We can therefore define which in general may depend on the system under study [15] , [26] . The change of α can have dramatic consequences for the long-term behaviour of systems ( Supplementary Figs S1–S4 and Supplementary Note 1 ). Dependence of α on δ / τ We now proceed to decrease τ . Some samples of x t are shown in Fig. 4a–c : the oscillations become faster and wider as τ decreases ( τ =0.6, 0.2 and 0.1 μs for Fig. 4a–c , respectively). We remark that the shorter the τ , the more closely the conditions for the applicability of the Wong–Zakai theorem [19] are met. One might expect that the circuit equation will follow the Stratonovich equation even more closely and thus, we shall expect no change with respect to the situation illustrated in Fig. 3 . However, as we can see in Fig. 4d–f , as τ decreases, the equilibrium position of the system moves back towards y =0. 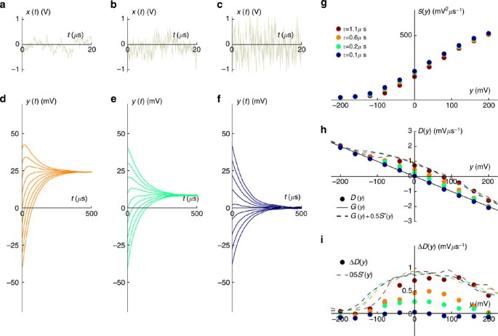Figure 4: Behaviour dependence on the noise correlation timeτ. (a–c) Samples of input noisesxtwithτ=0.6, 0.2 and 0.1 μs respectively for (a), (b) and (c). (d–f) Average of 1,000 trajectories for various initial conditions with τ=0.6, 0.2 and 0.1 μs respectively for (d), (e) and (f); there is a shift of the equilibrium towardsy=0. (g) DiffusionS(y). (h) DriftD(y) (dots), harmonic restoringG(y) (solid line) andG(y)+0.5S′(y) (dashed lines). (i) the ratio between the noise-induced extra-drift ΔD(y) and 0.5S′(y) clearly varies as a function of τ. Figure 4: Behaviour dependence on the noise correlation time τ . ( a – c ) Samples of input noises x t with τ =0.6, 0.2 and 0.1 μs respectively for ( a ), ( b ) and ( c ). ( d – f ) Average of 1,000 trajectories for various initial conditions with τ=0.6, 0.2 and 0.1 μs respectively for ( d ), ( e ) and ( f ); there is a shift of the equilibrium towards y =0. ( g ) Diffusion S ( y ). ( h ) Drift D ( y ) (dots), harmonic restoring G ( y ) (solid line) and G ( y )+0.5 S ′( y ) (dashed lines). ( i ) the ratio between the noise-induced extra-drift Δ D ( y ) and 0.5 S ′( y ) clearly varies as a function of τ. Full size image Clearly, this behaviour is not the result of a varying feedback; in fact, F ( y ) is the same in all the cases, as evidenced by the fact that the experimental values of S ( y ) do not vary significantly (symbols in Fig. 4g ). Instead, it comes from the fact that, as τ decreases, D ( y ) (symbols in Fig. 4h ) tends to G ( y ) or, equivalently, Δ D ( y ) (symbols in Fig. 4i ) tends to 0. Using Equation 6 and S ′( y ) (dashed line in Fig. 4i ), it is possible to calculate α , which goes from 0.5 to 0 as τ decreases. Thus, the SDE (4) shifts from obeying the Stratonovich calculus ( α =0.5 for τ =1.1 μs) to obeying the Itô calculus (α=0 for τ=0.1 μs). As we have remarked in the Introduction, such a Stratonovich-to-Itô transition can have a dramatic effect on the long time dynamics of the system, for example, altering the system’s equilibria as shown in Fig. 4d–f . In fact, this transition occurs because of the delay in the feedback. We measured the feedback delay in the circuit for the data shown in Fig. 2 and Fig. 3 to be δ =0.4 μs (Methods). The dots in Fig. 5 represent α as a function of δ / τ . The transition occurs as τ becomes similar to δ , that is, δ / τ ≈1. In order to verify the dependence of α on the ratio δ / τ , we performed additional experiments keeping τ =0.4 μs fixed and varying δ . For this purpose, we added a delay line in the feedback branch of the circuit so that we could adjust δ =0.9–5.4 μs (Methods). The resulting values of α are plotted in Fig. 5 as squares and are in good agreement with the theoretical prediction given by Equation 8. We further verify the validity of Equation 8 with numerical simulations of various systems ( Supplementary Figs S1–S4 and Supplementary Note 1 ). 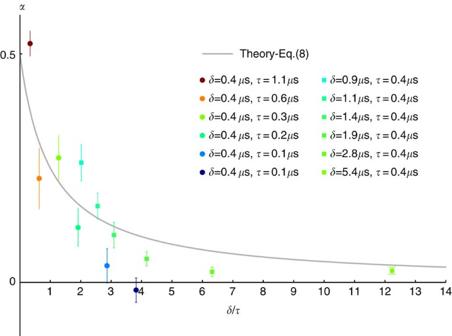Figure 5: Dependence ofαonδ/τ. αvaries from 0.5 (Stratonovich integral) to 0 (Itô integral) asδ/τincreases. The solid line represents the results of the theory (Equation 8); the dots represent the values ofαfor fixedδ=0.4 μs and varyingτ(Fig) and the squares for fixedτ=0.4 μs and varyingδ. The error bars represent one standard deviation obtained by repeating the experimental determination of the ratioδ/τ10 times. Figure 5: Dependence of α on δ / τ . α varies from 0.5 (Stratonovich integral) to 0 (Itô integral) as δ / τ increases. The solid line represents the results of the theory (Equation 8); the dots represent the values of α for fixed δ =0.4 μs and varying τ ( Fig ) and the squares for fixed τ =0.4 μs and varying δ . The error bars represent one standard deviation obtained by repeating the experimental determination of the ratio δ / τ 10 times. Full size image Mathematical analysis In order to gain a more precise mathematical understanding of this Stratonovich-to-Itô transition, we consider the following family of delayed SDEs where is a sufficiently regular noise with correlation time τ and the feedback is delayed by δ . Studying the limits where δ,τ→0 under the condition δ/τ≡constant, we recover the SDE (2) with This result holds for all SDEs with delayed feedback; the details of the proof are given in the Methods and in the Supplementary Note 2 . Figure 5 shows the agreement between Equation 8 (grey line) and the experimental data as a function of δ / τ (symbols). The reason for the Stratonovich-to-Itô transition captured in Equation 8 lies in the underlying dynamics of the system modelled by the SDE (4). For most real physical, chemical, biological and economic phenomena such microscopic dynamics are either too complex to be modelled or simply experimentally inaccessible. This justifies the need to resort to effective models, for example, SDEs (see Supplementary Figs S1–S4 and Supplementary Note 1 for some potential examples from biology, economics and physics). For this work we have chosen a model system, that is, an electric circuit, that gives us complete access to the underlying dynamics. We are therefore able to track down the observed Stratonovich-to-Itô transition to the fact that the feedback is not instantaneous but involves a delay. The fact that this transition occurs as τ becomes similar to δ , that is, δ / τ ≈1 ( Fig. 5 ) can be qualitatively explained considering that, if δ=0, there is a correlation between the sign of x and the time-derivative of F ( y ), which is the underlying reason why the process converges to the Stratonovich solution [19] ; however, if , this correlation disappears, effectively randomizing the time-derivative of F ( y ) with respect to the sign of x and leading to a situation where the system loses its memory. The result in Equation 8 can be generalized to systems with many state variables, even when the delay and the correlation time for each state variable of the system are not the same ( Supplementary Note 3 ). In general, within a given system there can be different values of α , and therefore different corresponding stochastic integral conventions. As in Equation 8, each value of α depends on the ratio between a feedback delay time and a noise correlation time. Our results show that the intrinsic ambiguity in the models of physical, biological and economic phenomena using SDEs with multiplicative noise can have concrete consequences. In particular, the stochastic integration convention needed to interpret an SDE correctly may vary with the parameters of the system. Notably, our result that a Stratonovich-to-Itô transition occurs if the delay in the feedback ( δ ) is longer than the correlation time of the noise ( τ ) has general applicability because instantaneous feedback and white noise are only mathematical approximations. The possibility of such a shift and of its consequences is worth exploring in the numerous cases where SDEs with multiplicative noise are routinely employed to predict the behaviour and evolution of complex physical, chemical, biological and economic phenomena. RC circuit The dynamical system employed in our experiments is an RC electric circuit. A noisy signal x t , which is generated by a function wave generator (Agilent 33250A) and pre-filtered by a low-pass filter to set the desired τ , drives the RC series. The system’s state y t is measured on the capacitor using a digital oscilloscope (Tektronix 5034B, 350 MHz bandwidth) at 10 6 samples per second, which are then subsampled before analysis. For the circuit with feedback, a high-speed low-noise analogue multiplier (AD835) is employed to multiply x t by the feedback signal (generated by amplifying y t and adding an offset) before applying it to the RC series. We measured the intrinsic delay of the circuit feedback branch (due to its finite bandwidth) applying a periodic deterministic signal and measuring the delay of the response. The additional delay line was realized by employing an analogue variable delay amplifier (Ortec 427A). Estimation of S ( y ) and D ( y ) In order to estimate diffusion S ( y ) and drift D ( y ) from an experimentally acquired time series, we use their definition [15] following a standard approach (see, for example, refs 27 , 28 ), which has also been applied to the stochastic analysis of electric circuits [29] . Letting the system evolve from an initial state y for an infinitesimal time-step, S ( y ) is proportional to the variance of the system’s state change (inset in Fig. 2c ) and D ( y ) to its average (inset in Fig. 2d ). S ( y ) and D ( y ) can be obtained from an experimental discrete time-series ( y 0 ,..., y N −1 ) sampling the output signal at intervals Δ t as and In Equations 9 and 10 Δ t should be chosen very carefully when fitting data from a process with several time scales to a homogenized low-dimensional model, as we do in this article [30] . In our case, Δ t should meet the condition , which warrants that the data are subsampled with respect to the fast time scales of the process we consider and therefore the estimation of the drift and diffusion of the homogenized low-dimensional model is correct [30] . Furthermore, Δ t should also be much smaller than the relaxation time of the system [25] . Both conditions are verified in the experiments presented in this article by subsampling the experimental data at Δ t =10 μs. Derivation of Equation 8 We study the solution of Equation 7, taking the limit in which δ,τ→0 at the same rate so that δ/τ stays constant. In order to deal with a sufficiently regular process, we take as a harmonic process [31] , letting , where is the stationary solution of the SDE where Γ and Ω are constants, W t is a Wiener process and τ is the correlation time for the Ornstein–Uhlenbeck process obtained by taking the limit Γ, Ω 2 →∞ while keeping constant. As τ→0, the rescaled solution of Equation 11, , converges to a white noise. We define the process by , and we write Equation 7 in terms of . Next, we expand about t to first order in δ and rewrite the resulting equation as a first-order system in , v , and z , where . We then consider the backward Kolmogorov equation associated with the resulting SDE, which gives the equation for the transition density . We can expand ρ in powers of the parameter , that is, . We use the standard homogenization method [32] to derive the backward Kolmogorov equation for ρ 0 [33] , that is, the equation for the limiting transition density ρ 0 as τ,δ→0 with δ/τ≡constant. Finally, we take the limit Γ,Ω 2 →∞ while keeping the ratio constant. The resulting backward Kolmogorov equation is and the associated (Itô) SDE is Mathematically, convergence of the Kolmogorov equations means convergence of infinitesimal operators (generators) of the diffusion processes defined by solving the associated SDE’s. It follows that the solutions converge in distribution to the solution of the limiting equation. The equation for α (Equation 8) follows straightforwardly by comparison of Equations 2 and 13. A more detailed derivation is provided in Supplementary Note 2. How to cite this article: Pesce, G. et al. Stratonovich-to-Itô transition in noisy systems with multiplicative feedback. Nat. Commun. 4:2733 doi: 10.1038/ncomms3733 (2013).